Genome-wide adaptive complexes to underground stresses in blind mole ratsSpalax The blind mole rat (BMR), Spalax galili , is an excellent model for studying mammalian adaptation to life underground and medical applications. The BMR spends its entire life underground, protecting itself from predators and climatic fluctuations while challenging it with multiple stressors such as darkness, hypoxia, hypercapnia, energetics and high pathonecity. Here we sequence and analyse the BMR genome and transcriptome, highlighting the possible genomic adaptive responses to the underground stressors. Our results show high rates of RNA/DNA editing, reduced chromosome rearrangements, an over-representation of short interspersed elements (SINEs) probably linked to hypoxia tolerance, degeneration of vision and progression of photoperiodic perception, tolerance to hypercapnia and hypoxia and resistance to cancer. The remarkable traits of the BMR, together with its genomic and transcriptomic information, enhance our understanding of adaptation to extreme environments and will enable the utilization of BMR models for biomedical research in the fight against cancer, stroke and cardiovascular diseases. The subterranean blind mole rat (BMR), Spalax galili , belongs to the Spalax ehrenbergi superspecies in the family Spalacidae, a clade of subterranean muroid rodents distributed in the Eastern Mediterranean and North Africa. BMRs are solitary mammals that spend their lives in underground burrows, which shelter them from most predators and climatic fluctuations. However, in this subterranean environment they are challenged by multiple stressors such as darkness, hypoxia, hypercapnia, energetic challenges during digging and increased exposure to pathogens [1] , [2] , [3] . Consequently, BMRs evolved multiple genetic adaptations to cope with these stresses. This has provided researchers with a unique evolutionary model for investigating stressful life underground. The BMR has been extensively studied genomically, proteomically and phenomically [1] , [2] , [3] , [4] , [5] , [6] , [7] , [8] , [9] , [10] , [11] , [12] , [13] , [14] , [15] , [16] , [17] , [18] , [19] , [20] , [21] , [22] , [23] , [24] , [25] , [26] , [27] , [28] , [29] , [30] , [31] , [32] , [33] , [34] , [35] (for full list of publications please refer to the online Spalax publication list: http://evolution.haifa.ac.il/index.php/28-people/publications/152-publication-nevo-spalax ). The lack of light in subterranean burrows presumably has triggered a complex mosaic of traits involving light perception, including severe ocular regression with a subcutaneous minute degenerated eye, coupled with the elaboration of photoperiodic perception [16] , [17] . The BMR has evolved a larger brain volume compared with that of rodents of similar body size because of the development of an expanded neocortex with developed vibrational, tactile, vocal, olfactory and magnetic (spatial) orientation systems replacing sight as well as the enlargement of the motor structures related to digging activity [18] , [19] , [20] , [21] , [22] , [23] . Most remarkably, the BMR has evolved physiological strategies to survive and carry out intense activities in a highly hypoxic and hypercapnic environment with wide fluctuations in oxygen concentration (O 2 as low as 7.2% and CO 2 as high as 6.1% were recorded in underground burrows [24] ). These adaptions include improved myocardial oxygen delivery and function [25] , adaptive heart and breathing frequencies [26] , high blood haemoglobin and haematocrit concentrations [27] , respiratory adaptations [28] , enlarged alveolar surface area and alveolar capillary volume [29] and increased tissue mitochondrial and capillary densities [29] , [30] . At the molecular level, a growing list of genes has been reported to underlie the BMR’s hypoxic tolerance [4] , [31] , [32] . For example, constitutively increased mRNA and protein expression levels (compared with rat) of myoglobin in muscle, neuroglobin in the brain and cytoglobin in fibroblast-like cells [31] were observed. BMR p53 has a substitution in a DNA-binding domain identical to a human tumour-associated mutation, which inhibits hypoxia-induced apoptosis in favour of cell cycle arrest [33] and necrosis. In addition, the BMR shows a striking resistance to cancer: not a single case of spontaneous tumour development was recorded among thousands of captive animals over a 40-year period, including animals over 20 years old that may be more vulnerable to cancer. Experiments using chemical carcinogens to induce tumour growth had negative results in BMR, while 100% of mice, rats and Acomys (an additional wild rodent species) developed tumours [34] . Moreover, in an in vitro system BMR fibroblasts were shown to inhibit growth and even kill cells from various human cancer cell lines [34] . Recent findings suggest that the unique BMR anticancer mechanism is mediated by an induction of the necrotic cell-death mechanism in response to hyperproliferation [35] . Here we report the sequencing and analysis of the BMR genome and transcriptome. Our results reveal the unique adaptive genomic features of the BMR, including high rates of DNA and higher RNA editing compared with that of the mouse and rat, lower rates of chromosome rearrangements, as well as an over-representation of SINE (short interspersed element) transposable elements, which is likely because of a novel response to hypoxia tolerance. In addition, our analysis of the BMR genome and transcriptome identifies the evolution of placenta-specific genes and revealed molecular adaptations involved in response to darkness, tolerance of hypercapnia and hypoxia, for example, by modifications of respiratory proteins, and resistance to cancer. The extreme adaptations and characteristics of the BMR, together with the reported genome and transcriptome, will empower future use of the BMR model for biomedical research in the fight against cancer, stroke and cardiovascular diseases. Genome assembly and annotation The DNA obtained from the brain of a female Spalax galili (a diploid with the chromosome number of 2 n =52) was sequenced using a whole-genome shotgun strategy utilizing Illumina sequencing technology. 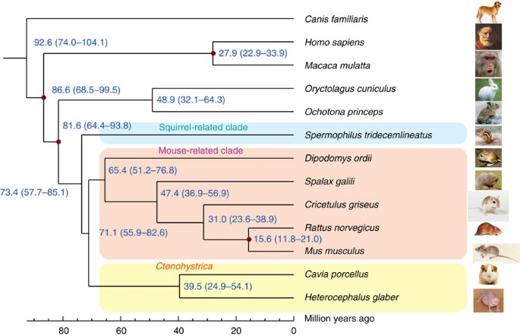Figure 1: BMR phylogeny and estimation of divergence times. The time of divergence (with error range shown in parentheses) of BMR and 12 other mammals based on orthologous proteins. Points of taxon divergence are shown in millions of years. Our result supports the division of rodents into three clades: the Mouse-related clade, Ctenohystrica (guinea pig and relatives) and the Squirrel-related clade70. Various insert size libraries were used to generate 392 Gbp of raw data, of which 259 Gbp (86 × coverage) of high-quality data were retained for assembly ( Supplementary Table 1 ). 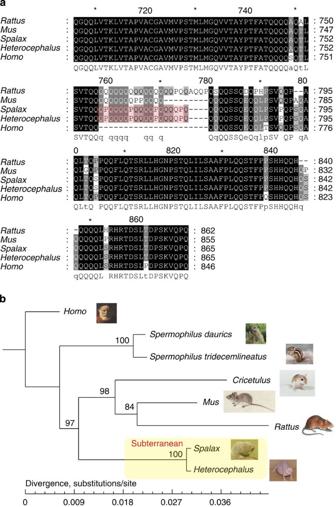Figure 2: Convergent evolution of BMR and NMR CLOCK proteins. (a) The Q-rich domain of BMR (Spalax) and NMR (Heterocephalus) CLOCK proteins compared with that of human (Homo), rat (Rattus) and Mouse (Mus). Red box indicated the expanded glutamine-rich area in BMR and NMR. (b) Phylogenetic tree of the CLOCK protein. The rooted tree describes the similarity relationships among the CLOCK proteins of BMR, NMR, mouse, rat, Ord's Kangaroo Rat (Dipodomys), thirteen-lined ground Squirrel (Spermophilus tridecemlineatus), Daurian ground squirrel (S. dauricus) and human (Homo). 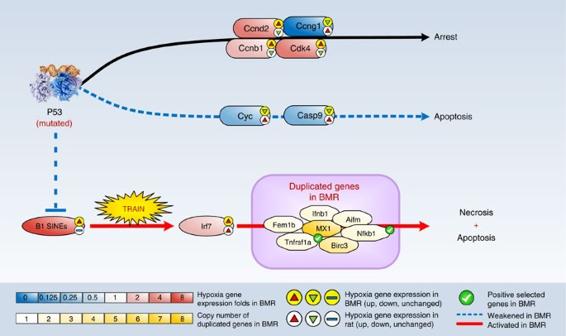Figure 3: BMR adaptive complex related with hypoxia tolerance and cancer resistance. The colours of elementsCcnd2,Ccng1,Ccnb1,Cdk4,Cyc,Casp9,Irf7and B1 SINEs depict expression fold changes according to RPKM, while colours ofMx1,Birc3,Ifnb1, A1fm1,Nfkb1,Tnfrsf1aandFem1Brepresent gene copy number amplification. The green check marks onTnfrsf1aandNfkb1indicate evidence of positive selection. Genome assembly using SOAPdenovo [36] as described [37] produced a final assembly of 3.06 Gbp, consistent with the kmer-based genome size estimation (~3.04 Gbp, Supplementary Table 2 , Supplementary Figs 1 and 2 ); the contig and scaffold N50s were 27.5 kbp and 3.6 Mbp, respectively ( Supplementary Table 3 ). The average GC content is 41.23%, comparable to the human genome [38] . To assess the quality of the assembly, BMR and rat transcriptome data generated for this study were mapped on our BMR assembly and the rat genome, respectively; on average, 81.5% of reads mapped to the BMR assembly, comparable to 82.1% that mapped to the rat. Transcriptome assembled contigs using Trinity [39] were mapped to the BMR genome. Of the 63.38 Mb contigs, 98.9% were covered by more than 90% coverage, suggesting the completeness of transcript representation in our assembly. Moreover, randomly selected 20-fold of paired-end reads from short insert size libraries were aligned to the assembly, and 92.75% were successfully mapped using BWA (Burrow-Wheeler Aligner, version 0.5.9-r16) [40] , giving a genome coverage of ~99.57%, suggesting our assembly covered most of the genome ( Supplementary Tables 4 and 5 ). We identified 3.26-M single-nucleotide polymorphisms (SNPs) and 627-K short InDels, the heterozygosis of SNP and InDel were estimated to be 0.11% and 0.02%, respectively, or 0.13% combined together. This is comparable to the human, but is higher than its relative, another subterranean rodent called the naked mole rat (NMR, Heterocephalus glaber ), which is proposed as naturally inbred because of its eusocial behaviour [41] . By analysing the context dependency of BMR SNPs, we found heavy reduction in SNPs because of CpG mutations compared with other mammals ( Supplementary Fig. 3 ). BMR also has a lower CpG observed/expected value compared with other mammals ( Supplementary Fig. 4 ) and a higher fraction of CpG dinucleotides concentrated in CpG islands as compared with the mouse or rat ( Supplementary Table 6 ). More details shown in Supplementary Note 1 . Reference-assisted chromosome assembly [42] reconstruction of predicted chromosome fragments (PCFs) of the BMR genome was performed using a threshold of 50 and 80 kbp to include syntenic fragments (SFs) in two independent reconstruction experiments, respectively ( Supplementary Note 2 and Supplementary Table 7 ). At 50 kbp resolution, 41 PCFs were recovered, covering 82.1% of the BMR genome, while at 80 kbp resolution, 36 PCFs were reconstructed, giving an overall genome coverage of 76.8%. These 36 PCFs contain 18 interchromosomal rearrangements of which 17 occurred in the Muridae lineage (mouse and rat) and one in the BMR lineage. The number of BMR scaffolds containing >1 SF was 25 (3.6%, 80 kbp resolution). These mainly represent BMR-specific chromosomal rearrangements, several chimeric scaffolds or, in some rare instances, misalignments between the BMR, mouse and human sequences. These scaffolds contain 27 potential evolutionary breakpoint regions. At 80 kbp resolution, our data indicate that the BMR genome evolved with the rate of at least 0.56 rearrangements after the split from a common ancestor with the mouse ~47.6 million years ago (MYA; www.timetree.org ; Supplementary Fig. 5 ). This rate is lower than the ~2.1 and ~1.9 rearrangements per million years (300 kbp resolution) in artiodactyl and primate genomes [43] , suggesting that a striking stability of the BMR chromosomal arms in evolution could compensate for a large number of chromosomal fusions and fissions observed in BMR chromosomal species and speciation. Repeats constitute 43.9% of the BMR genome, with retrotransposons being the most prevalent transposable elements (32.5% of the genome). Interestingly, the proportion of SINEs (11.8%) in BMR is more similar to that in the human genome (13.7%), and much higher than in other sequenced rodents (6.5%, 5.6% and 5.6% in the mouse, rat and NMR [41] , respectively). B1, B2 and B4 are the three most abundant SINEs (10% of the genome) in the BMR assembly, indicating a BMR-specific expansion of these transposable elements compared with mouse, rat, NMR and human ( Supplementary Figs 6–8 , Supplementary Table 8 , Supplementary Data 1–3 ). The functional role of B1, B2 and B4 SINEs in mouse has been intensively investigated. B1 and B2 were shown to be stress-inducible factors in the ischaemic brain [44] . In addition, upregulation of B2 SINE RNA downregulates transcription in response to heat shock in mouse [44] , [45] , [46] . B2 can induce polymorphic expression of the 5-aminolevulinic acid synthase 1 ( ALAS1 ) gene, the key to nonerythroid haem homeostasis and fundamental in respiration, drug metabolism and cell signalling [47] . Therefore, the over-representation of B1, B2 and B4 SINEs in the BMR genome might reflect exposure to hypoxic stresses in the underground environment. In particular, we found that the B1 SINE repeat showed high upregulation (see below) under severe hypoxia in the BMR brain. A similar mode of regulation was reported for human Alu SINEs that were shown to be transcriptionally upregulated under hypoxic conditions, presumably contributing to genomic instability in tumours [48] . Gene annotation and molecular phylogeny We obtained a reference gene set that contained 22,168 coding genes in the BMR genome by combining homologous searching, transcriptome evidence and de novo prediction ( Supplementary Note 3 ; Supplementary Tables 9 and 10 ). Of the predicted genes, 19,730 (89%) were recovered by the RNA-seq data. Among the reference genes of BMR, orthologues with other animals showed highest similarity between the BMR and Chinese hamster ( Cricetulus griseus ; Supplementary Table 11 , Supplementary Fig. 9 ). We inferred 12,767 gene families ( Supplementary Fig. 10 ) and constructed a phylogenetic tree from 1,583 single-copy orthologues. As shown in Fig. 1 , the BMR was placed within Rodentia and diverged from the ancestor of rats, mice and Chinese hamster ( C. griseus ) ~47 MYA, consistent with a previous study [1] . The common ancestor of the BMR, mouse, rat and Chinese hamster separated from a lineage leading to NMR ~71 MYA. In comparison with several other sequenced mammalian genomes, we estimated that 139 gene families showed expansion and 50 gene families showed contractions in the BMR ( Supplementary Data 4 and 5 ; Supplementary Fig. 11 ). BMR- and NMR-specific genes are shown in Supplementary Data 6 and 7 and Supplementary Table 12 . We also detected 35 lost genes ( Supplementary Table 13 ) and 259 pseudogenes ( Supplementary Data 8 , Supplementary Tables 14 and 15 ), as well as 48 positively selected genes ( Supplementary Data 9 , Supplementary Tables 16 and 17 ) during BMR evolution, which altogether may underlie the physiological adaptations of the BMR to its stressful underground niche. Copy numbers of certain cancer-related genes in BMR, NMR, mouse and rat are shown in Supplementary Data 10 . Figure 1: BMR phylogeny and estimation of divergence times. The time of divergence (with error range shown in parentheses) of BMR and 12 other mammals based on orthologous proteins. Points of taxon divergence are shown in millions of years. Our result supports the division of rodents into three clades: the Mouse-related clade, Ctenohystrica (guinea pig and relatives) and the Squirrel-related clade [70] . Full size image One outstanding issue in the evolution of murid reproduction is the timing of diversification of murid-specific genes expressed solely in the placenta (cathepsins, prolactins, pregnancy-specific glycoproteins and syncytins) [49] . We sequenced the transcriptome of the placenta in BMR and queried the BMR genome using rodent transcripts ( Supplementary Note 4 ; Supplementary Table 18 ). We identified 13 prolactins, 6 pregnancy-specific glycoproteins and 4 placental cathepsins. These numbers are intermediate between murids and NMR ( Supplementary Table 19 and Supplementary Figs 12 and 13 ), implying that these families had started to diversify before the origin of Muroidea ~47 MYA [50] . In addition, we identified two murid-specific syncytins ( Syna and Synb ), both of which are not present in the NMR. This is potentially because of differences in placental morphology. Extensive DNA and RNA editing increases adaptive potentials Increase in genomic diversity may reinforce the adaptation to subterranean lifestyle. DNA and RNA editing of retroelements enhances intra- and interspecies diversity. We screened the BMR genome and transcriptome for these, making BMR one of the first organisms to be comprehensively analysed for both types of editing, preceded only by human and mouse [51] . First, we detected DNA editing of retroelements across the assembly. The BMR genome contains one APOBEC3 ( A3 ) gene, whose product can introduce a series of C to U mutations into the negative strand of nascent retroelement DNA. Generation and analysis of paired alignments within LTR retrotransposon families revealed numerous retroelements containing clusters of G to A mutations, signs of DNA editing by A3 (2,459 elements, 23,853 edited nucleotides). BMR A3 , identical in protein sequence to its murine counterpart, is also identical in its preference for the G xA motif in LTR retroelement-editing sites [52] . Another trait shared by the BMR and murine genomes is a strong signal of editing in the active Intracisternal A-type particle retroelements [53] . For detailed information please refer to Supplementary Note 5 , Supplementary Tables 20–23 , Supplementary Data 11–15 and Supplementary Figs 14–20 . Next, we detected RNA editing making use of transcriptome reads obtained from BMR and rat hypoxia samples ( Supplementary Figs 21–33 ). A-to-I RNA editing is more prevalent in primates than in rodents [54] and catalysed by adenosine deaminases acting on RNA (ADAR) enzymes. Abundance of similar SINEs in a genome increases the chance of two similar and reversely oriented elements to reside next to each other [55] . When transcribed, they are likely to form a double-stranded RNA structure, the preferred substrate for ADAR. We mapped RNA reads to the assembled genome and found mismatches in 257,094 SINE elements. As RNA editing tends to come in clusters, we searched for these and detected 19,714 SINEs with at least four mismatches of the same type, with a total of 113,338 AG/TC-editing sites, containing the ADAR sequence motif, supporting their authenticity. Strikingly, the number of editing sites was >107 times greater than the number of the control mismatch clusters (G to A/C to T). A similar comparison to rat yielded only a 14:1 ratio between editing and control sites. Together with previous analyses of mouse RNA editing [55] , [56] , we conclude that the BMR’s RNA-editing occurrence is higher than those of both the rat and mouse. We predict that a relatively large number of lineage-specific RNA-editing events take place in many BMR genes, contributing to its unique adaptation, without necessitating mutations in the genome. Adaptation to darkness The lack of visible light underground triggered a complex degradation of the eye in the BMR involving drastic ocular regression with a small degenerate subcutaneous eye and a simultaneous elaboration of circadian rhythm perception. Of the 259 pseudogenes found in the BMR genome, there are 22 genes involved in the visual system ( Supplementary Table 15 ). Fifteen of these visual system pseudogenes contain no alternative splicing forms to avoid the mutation sites and are likely complete pseudogenes. A comparison of the BMR gene families with those of other species (human, monkey, rabbit, rat, mouse, NMR and dog) indicated a contraction in the beta/gamma crystalline gene family ( P value=0.047), potentially linked with the BMR’s degradation of vision. This confirms our previous results [57] that transgenic mice carrying the BMR crystallin gene selectively lose lens activity after 13 days of embryogenesis. The circadian rhythm of the BMR has been previously studied and genes involved were identified [58] , [59] , [60] . Multi-alignments of the protein sequences of circadian genes revealed that both BMR and NMR CLOCK proteins have an expanded Q-rich region compared with that of the human and mouse, and are different in amino-acid composition from that of the rat [58] ( Fig. 2a ). The phylogenetic tree indicates that the BMR and the NMR CLOCK proteins display a higher similarity in amino-acid composition, despite being phylogenetically distant ( Fig. 2b ). Since the glutamine-rich area is assumed to be involved in circadian rhythmicity [58] , the similarity in amino-acid composition of the BMR and NMR Clock genes may indicate convergent evolution by these subterranean animals. Figure 2: Convergent evolution of BMR and NMR CLOCK proteins. ( a ) The Q-rich domain of BMR ( Spalax ) and NMR ( Heterocephalus ) CLOCK proteins compared with that of human ( Homo ), rat ( Rattus ) and Mouse ( Mus ). Red box indicated the expanded glutamine-rich area in BMR and NMR. ( b ) Phylogenetic tree of the CLOCK protein. The rooted tree describes the similarity relationships among the CLOCK proteins of BMR, NMR, mouse, rat, Ord's Kangaroo Rat ( Dipodomys ), thirteen-lined ground Squirrel ( Spermophilus tridecemlineatus ), Daurian ground squirrel ( S. dauricus ) and human ( Homo ). Full size image In addition, the glial cell line-derived neurotrophic factor family has expanded in BMR because of multiple duplications of the gene Gfra1 . As the BMR brain is twice as large as that of a rat with similar body size [21] , [22] , [23] , and since Gfra1 can serve as a potent neuronal survival factor [61] , its over-representation may have contributed to the enlargement of the motor structures and somatosensory system in the BMR brain, enabling highly developed digging activity and sense physiology to replace sight [18] , [19] , [20] . Adaptation to hypercapnia and hypoxia Transcriptome analysis ( Supplementary Note 6 , Supplementary Data 16 and 17 , Supplementary Figs 34–42 and Supplementary Tables 24 and 25 ) revealed an upregulation of BMR genes after experimental hypoxia, including known HIF-1 targets, such as hexokinase ( Hk1 ), adrenomedullin ( Adm ), macrophage migration inhibitory factor ( Mi f), ankyrin repeat domain-containing protein 37 ( Ankrd37 ) [6] , [62] , secretogogin ( SCGN ), neuromedin-B ( NMB ) and cocaine-and-amphetamine-regulated transcript ( CART ). GO analysis ( Supplementary Data 18 ) indicated that hypoxia-upregulated genes were enriched in terms related to cellular defense, response to steroid hormone stimulus, ribosome biogenesis, mitochondrial ribosome, RNA splicing, cytoskeleton, regulation of circulation and blood pressure, regulation of appetite, and regulation of circadian rhythms. At the same time, hypoxia-downregulated genes were enriched in terms related to neuron morphogenesis, intracellular protein transport, transmission of nerve impulses, phosphate metabolic processes, regulation of cell motion, regulation of protein kinase activity and nuclear protein import. Some of these processes have not been reported before as being enriched in BMR under conditions of hypoxia. As BMR p53 has a substitution, enabling cells to escape hypoxia-induced apoptosis in favour of a reversible cell cycle arrest [33] , we compared expression levels of 57 BMR and rat orthologues involved in the p53 signal pathway ( Supplementary Data 19 ). Eight p53 target genes were found to be differentially regulated by hypoxia in BMR and rat ( Supplementary Data 20 ). Sestrin ( Sesn1 ), cyclin G ( Ccng1 ), Mdm2 , CytC and Casp9 were downregulated in BMR but upregulated in rat, while Ccnb1 , cyclin D ( Ccnd2 ) and CDK 4/6 ( Cdk4 ) were upregulated in BMR but downregulated in rat ( Fig. 3 ). Since the induction of CytC is a reflection of oxidative stress and the upregulation of Casp9 may point to the activation of mitochondrial apoptosis, we assume that p53 in BMR downregulates apoptosis to avoid excessive cell loss under hypoxic conditions. Our analysis results contradict previous results [9] , [32] on the upregulation of Mdm2 in the brain; instead, we found downregulation. This discrepancy might be explained by the difference in platforms and applied analysis techniques. Figure 3: BMR adaptive complex related with hypoxia tolerance and cancer resistance. The colours of elements Ccnd2 , Ccng1 , Ccnb1 , Cdk4 , Cyc , Casp9 , Irf7 and B1 SINEs depict expression fold changes according to RPKM, while colours of Mx1 , Birc3 , Ifnb1 , A1fm1, Nfkb1 , Tnfrsf1a and Fem1B represent gene copy number amplification. The green check marks on Tnfrsf1a and Nfkb1 indicate evidence of positive selection. Full size image The B1 SINE repeat showed significant transcriptional upregulation in hypoxia in BMR, but not in rat ( Supplementary Note 7 ; Supplementary Table 26 ; Supplementary Fig. 43 ). Interestingly, it has recently been shown [63] that p53 negatively controls B1 SINE repeat expression in normal mammalian cells and that weak p53 control of this expression can lead to massive transcription of B1 and B2 SINEs accompanied with activation of an interferon response (TRAIN ‘transcription of repeats activates interferon’ phenomenon). Consistently, our RNA-Seq data indicate that several interferon regulatory factors, implicated in the TRAIN response, are upregulated in BMR but not in rat under hypoxic conditions ( Fig. 3 ). As p53 in BMR is known to have a tumour-like substitution [33] , [64] , it may be that it has a weaker SINE-inhibitory effect than rat p53, thus enabling activation of the TRAIN. Several types of L1 elements demonstrate significant upregulation of expression in BMR under 3% of oxygen ( Supplementary Fig. 44 ). Together with B1 upregulation, this fact could be interpreted as follows: the L1 elements facilitate the genomic propagation and insertion of non-autonomous SINE elements because L1 (LINE-1) retrotransposons are encoding reverse transcriptase (RT) proteins. This L1-derived RT is used by SINE B1 retrotransposons (that do not encode RT) for their retrotransposition [65] . The combination of ‘weak’ p53, permitting transcription of SINEs and L1 (source of RT) under hypoxic conditions, and frequent exposure to hypoxic stress creates conditions facilitating amplification of SINEs and provides a plausible explanation for high abundance of SINEs in the genome BMR vis-à-vis rodents living under normal conditions. We inferred the genomic organizations of alpha and beta hemoglobin (HB) gene clusters from BMR (scaffolds 104 and 635, respectively; Supplementary Note 8 ; Supplementary Figs 45 and 46 ). BMR features a mutation in the proton-gated nociceptor sodium channel Nav1.7 (gene name Scn9a ), which results in the replacement of a highly conserved positively charged amino-acid motif (KKV) in domain IV of Nav1.7 by the negatively charged EKD motif. Interestingly, a related mutation, resulting in a negatively charged EKE motif, was found in the NMR Nav1.7. This mutation is thought to attract protons, thereby blocking the channel and thus protecting the NMR tissue from hypercapnia-induced acid pain [66] . A phylogenetic interpretation of Nav1.7 sequence evolution in mammals ( Fig. 4 ) suggests that the pain-blocking mutation is an adaptive trait, which has arisen independently in hypercapnia-exposed species by convergent evolution. 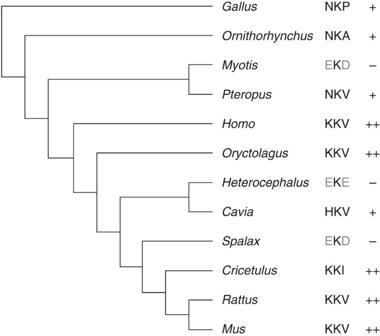Figure 4: Evolution of the adaptive amino-acid sequence motif from the sodium channel nociceptor protein Nav1.7 in mammals. Note the negative net charge of the motif (as indicated by + or −) in the hypercapnia-exposed BMR (Spalax), NMR (Heterocephalus) and the cave microbat (Myotis). The adaptive trait, which confers resistance to acidosis pain, has evolved by convergence in the three distantly related hypercapnic animal lineages. Figure 4: Evolution of the adaptive amino-acid sequence motif from the sodium channel nociceptor protein Nav1.7 in mammals. Note the negative net charge of the motif (as indicated by + or −) in the hypercapnia-exposed BMR ( Spalax ), NMR ( Heterocephalus ) and the cave microbat ( Myotis ). The adaptive trait, which confers resistance to acidosis pain, has evolved by convergence in the three distantly related hypercapnic animal lineages. Full size image Analyses of HB-coding sequences appear to confirm the uniqueness of BMR with respect to its embryonic haemoglobin gamma (HBG) component by revealing a comparatively fast rate of HBG sequence evolution and evidence of an elevated non-synonymous to synonymous substitution ratio, indicative of positive Darwinian selection ( Supplementary Figs 47 and 48 ). Three additional potentially reactive Cys residues in helices A, B and D of the BMR HBG T1 and T2 paralogues may in fact protect the embryonic globin from oxidation to the non-functional metHB (Fe 3+ ) form, as recently reported for Cys-enriched HBB haplotypes in mouse [67] . The cysteine content could also affect redox reactions and HB-mediated oxidative or nitrosative stress response [68] . We found that NMR, not BMR, adult HBA features a mutation (Pro(44)>His(44)), which is located in the switch region of the globin and affects interaction with His(97) of the HBB chain. It is therefore tempting to speculate that the His(44) amino-acid replacement in HBA, commonly observed in the two hystricomorphs NMR and Cavia porcellus , has facilitated an evolutionary adaptation of these taxa to hypoxic conditions, one in underground dwellings and the other in high-altitude habitats. Increased mRNA and protein expression levels observed in potentially hypoxia-adaptive genes in BMR versus rat are complemented by changes on the genic level: for example, Vegfb (Vascular endothelial growth factor B) has four copies in BMR. As growth factors regulate cell growth and division, Vegfb plays a significant role in the survival of blood vessels [69] and may therefore contribute to BMR’s adaptation to hypoxia. Cancer resistance BMR is resistant to both spontaneous cancer [35] as well as the induction of tumours by chemical carcinogens [34] . This may be because of the unique tumour suppression mechanism in which necrosis plays a major role as opposed to apoptosis normally used in many organisms. Necrosis in BMR cells is triggered by a release of interferon-beta in response to the overproliferation of cells [35] . Our analysis of the BMR genome showed that Ifnb1 , the gene encoding interferon-β1, underwent a duplication event in the BMR when compared with mouse, rat and NMR. These observations fit the following model. Acquisition of ‘weakened’ p53 by BMR, presumably as an adaptation to hypoxia, resulted in reduction of its tumour suppressor activity. A strong TRAIN-mediated suicidal interferon response enabled by the increased gene dosage of Ifnb1 is likely to be a highly effective compensatory mechanism that complemented insufficient p53-mediated tumour suppression. The Mx1 genes from the interferon signalling pathway, and multiple genes involved in regulation of cell death and inflammation ( Nfkb , Tnfrsf1a , Birc3 , Fem1b and Aifm1 ), also underwent expansion in the BMR ( Supplementary Data 10 ). Furthermore, three genes involved in necrosis and inflammation ( Tnfrsf1a , Tnfsf15 and Nfkb1 ) show evidence of positive Darwinian selection ( Supplementary Tables 20 and 21 , Fig. 3 ). This analysis indicates that BMRs may have evolved a cancer-resistance mechanism relying on heightened immunoinflammatory response via gene amplification within the interferon-β1 pathway. BMR has evolved adaptive complexes to cope with the stressful underground environment, making it an excellent model for studying adaptive evolution, including regressive and progressive, convergent and divergent evolutionary regimes. For example, darkness caused the BMR to undergo regressive (blindness) and progressive (photoperiodic perception) evolution. Convergent adaptations for hypercapnia and acidosis tolerance in BMR, NMR and bat were observed, while BMR and NMR followed divergent strategies in oxygen supply by respiratory proteins ( Supplementary Fig. 49 ) and in resistance to cancer. We observed that various types of transposable elements underwent expansions in different mammalian lineages, such as the increased copy number of B1/B2 in BMR, ID elements in rats and B4 in Jaculus jaculus . Whether these expansions were adaptive and what the evolutionary pressures associated with them were, are poorly understood. Our finding that SINE B1/B2 elements underwent expansion in Spalax , and the increase in these elements’ activity during hypoxia associated with the unique anticancer adaptation provides an insight into evolutionary forces shaping the transposon landscape in the Spalax genome. The most interesting story was shown in Fig. 3 . It is possible that the unique mutation on BMR p53 leads to different transcriptomic regulation patterns of several p53 target genes upon hypoxia. The expansion of B1 SINE repeats in BMR, and the significant upregulation of their expression upon hypoxia, coupled with the upregulation of Irf7 in BMR but not in rat, indicate that the BMR p53 is ineffective in suppressing B1 SINE expression, leading to activation of the TRAIN mechanism. Since normal p53 plays the key role in the accumulation of senescent cells which contribute to the aging phenotype, we speculate that weak/mutated BMR p53, does not efficiently send cells to senescence and fails to suppress SINE expression and subsequent TRAIN. This results in the eradication of those cells, which in normal mouse/rat would become senescent. In addition, in the downstream of IRF7 , multiple genes involved in the regulation of necrosis and inflammation, including genes Ifnb1 , Mx1 , Nfkb , Tnfrsf1a , Birc3 , Fem1b and Aifm1 , underwent duplication events in BMR compared with mouse, rat and NMR, and genes such as Tnfrsf1a and Nfkb1 also show evidence of positive selection, further emphasizing that the BMR may have evolved a unique mechanism heightening necrosis and immunoinflammatory responses to partly replace apoptosis, which contribute to its remarkable hypoxia tolerance, cancer resistance and anti-aging. The sequencing and analysis of the BMR genome and transcriptome here could open vast vistas of theoretical and applicative research programmes that will highlight how system evolution operates in nature and how it could be harnessed to cure urgent human medical challenges to support life. Sample collection All animal protocols were approved by the Institutional Ethics Committee. Spalax galili were captured in the field and housed under ambient conditions in individual cages in the Animal Facility of the Institute of Evolution, University of Haifa, with free access to vegetable and fruit food at 21–23 °C in a 12:12 light–dark cycle. Animals were killed with a lethal inhalation anaesthesia agent (isoflurane). DNA used for genome sequencing was isolated from the whole brain of an adult female individual. The hypoxia experiments were conducted in a closed cage using the precise oxygen percentage in a balloon with the appropriate percentage from a reliable company. RNA used for hypoxia transcriptome sequencing was extracted from the whole brain. Genome sequencing We applied whole-genome shotgun sequencing using the Illumina HiSeq 2000 to sequence the genome of BMR. In order to reduce the risk of non-randomness, 14 paired-end libraries, with insert sizes of about 250, 500, 800 bp, 2, 5, 10 and 20 kbp, were constructed. In total, we generated about 392.79 G of data, of which 259.65 G (86 × coverage) were retained for assembly after filtering out low quality and duplicated reads. Genome assembly The BMR genome was assembled de novo by SOAPdenovo v2.04.4. First, by splitting the reads from short insert size libraries (250~500 bp) into 51-mers and then merging the 51-mers, we constructed the de Bruijn graph. Second, contigs that exhibit unambiguous connections in de Bruijn graphs were collected. Third, the paired-end information was subsequently used to link contigs into scaffolds, step by step, from short insert sizes to long insert sizes. In the last step, some intrascaffold gaps were filled by local assembly using the reads in a read-pair, where one end uniquely aligned to a contig, while the other end was located within the gap. The final total contig size and N50 were 2.91 Gbp and 27.5 kbp, respectively. The total scaffold size and N50 were 3.06 Gbp and 3.6 Mbp, respectively. Chromosome fragments We applied reference-assisted chromosome assembly to reconstruct PCF of the BMR genome. The BMR scaffolds larger than 10 kbp in size were aligned against the mouse (mm9; reference) and human (hsg37; outgroup) genomes using SatsumaSynteny [43] programme. We used BWA to map the BMR mate-pair reads to BMR scaffolds. A minimum size of 50 and 80 kbp for SFs was used in two independent reconstruction experiments. Gene annotation We predicted the protein-coding genes in BMR using a combination of homology-based and de novo methods, as well as transcript evidence. For the homology-based prediction, human (Ensembl release 64), mouse (Ensembl release 64), rat (Ensembl release 64) and NMR proteins [41] were collected and mapped on the genome using TblastN. Then, homologous genome sequences were aligned against the matching proteins using Genewise to define gene models. For de novo predictions, Augustus, GlimmerHMM, SNAP and Genscan were employed to predict coding genes. Parameters were trained based on the predicted genes from searching homologous and high-confidence transcriptomes. In addition, RNA-seq data generated for this study were mapped to the genome using Tophat, and transcriptome-based gene structures were obtained by cufflinks ( http://cufflinks.cbcb.umd.edu/ ). Finally, all lines of gene evidence were combined together using GLEAN ( http://sourceforge.net/projects/glean-gene/ ). For genes that were predicted solely ab initio , only those with transcriptome coverage more than 50% or RPKM higher than 5 were retained for further analysis. We obtained a reference gene set that contained 22,168 genes for the BMR. Phylogenetic relationship We constructed a phylogenetic tree of the BMR and other sequenced rodents and mammals, including Chinese hamster ( Cricetulus griseus ), rat ( Rattus norvegicus ), mouse ( Mus musculus ), Ord's kangaroo rat ( Dipodomys ordii ), lesser Egyptian jerboa ( Jaculus jaculus ), guinea pig ( Cavia porcellus ), NMR ( Heterocephalus glaber ), thirteen-lined ground squirrel ( Spermophilus tridecemlineatus ), European rabbit ( Oryctolagus cuniculus ), American pika ( Ochotona princeps ), monkey ( Macaca mulatta ), human ( Homo sapiens ) and dog ( Canis familiaris ). Single-copy orthologous gene families (1,583) were used to construct the phylogenetic tree. CDS sequences from each single-copy family were aligned, guided by MUSCLE alignments of protein sequences and concatenated to one super gene for each species. Codon 1, 2 and 1+2 sequences were extracted from CDS alignments and used as input for building trees, along with protein and CDS sequences. Then, RaxML was applied to build phylogenetic trees under GTR+gamma for nucleotide sequences and JTT+gamma model for protein sequences. We used 1,000 bootstrap replicates to assess the branch reliability in RaxML. Placenta transcriptome sequencing We extracted and isolated RNA from the villous portion of the term placenta of two species of the BMR, S. galili (ID: R1280) and S. carmeli (ID: R1284). Library preparation and sequencing were performed by Expression Analysis Inc. (Durham, NC, USA) using Illumina HiSeq 2000 platform. Illumina sequencing was paired-end with read lengths of 100 bp. Hypoxia transcriptome sequencing For BMR, the set of samples includes two samples under 21% O 2 , one sample under 14% O 2 , one sample under 10% O 2 , two samples under 6% O 2 and one sample under 3% O 2 . For Rat, the set of samples includes one sample under 21% O 2 , one sample under 14% O 2 , one sample under 10% O 2 and two samples under 6% O 2 , RNA samples were abstracted from the whole brain. For each sample, an RNA sequencing library was constructed using the Illumina mRNA-Seq Prep Kit. Paired-end RNA-seq libraries were prepared following Illumina’s protocols and sequenced on the Illumina HiSeq 2000 platform. How to cite this article: Fang, X. et al . Genome-wide adaptive complexes to underground stresses in blind mole rats Spalax . Nat. Commun. 5:3966 doi: 10.1038/ncomms4966 (2014). Accession codes: The blind mole rat ( Spalax galili ) whole-genome shotgun projects have been deposited in DDBJ/EMBL/GenBank nucleotide core database under the accession code AXCS00000000 . All short read data have been deposited in DDBJ/EMBL/GenBank Short Sequence Read Archive under the accession code SRA096441 . Raw sequencing data of transcriptomes have been deposited in the Gene Expression Omnibus as under the accession code GSE49485 .